Lysine methylation of VCP by a member of a novel human protein methyltransferase family Valosin-containing protein (VCP, also called p97) is an essential and highly conserved adenosine triphosphate-dependent chaperone implicated in a wide range of cellular processes in eukaryotes, and mild VCP mutations can cause severe neurodegenerative disease. Here we show that mammalian VCP is trimethylated on Lys315 in a variety of cell lines and tissues, and that the previously uncharacterized protein METTL21D (denoted here as VCP lysine methyltransferase, VCP-KMT) is the responsible enzyme. VCP methylation was abolished in three human VCP-KMT knockout cell lines generated with zinc-finger nucleases. Interestingly, VCP-KMT was recently reported to promote tumour metastasis, and indeed, VCP-KMT-deficient cells displayed reduced growth rate, migration and invasive potential. Finally, we present data indicating that VCP-KMT, calmodulin-lysine methyltransferase and eight uncharacterized proteins together constitute a novel human protein methyltransferase family. The present work provides new insights on protein methylation and its links to human disease. Protein methyltransferases (MTases) modify a wide range of cellular proteins, with lysine and arginine being the predominant acceptor sites [1] . Protein methylation can be dynamic and serve regulatory purposes, or it can be static and function as an expansion of the amino-acid repertoire. Most MTases use S -adenosyl methionine (SAM) as methyl donor, and the human genome encodes over 200 putative SAM-dependent MTases, most of which remain uncharacterized [2] . The majority of these MTases belongs to either the SET domain family or to the seven β-strand superfamily, also designated 'Class I MTases' [2] , [3] . Most characterized lysine-specific MTases are SET domain proteins acting primarily on histones, but a few lysine-specific protein MTases have also been found in Class I. In humans, these are the histone-specific MTase DOT1L [3] and the calmodulin-specific MTase CaM-KMT [4] ; in addition, human METTL10 is a likely ortholog of yeast See1, which methylates elongation factor 1A [5] . The MTases responsible for many lysine methylations remain elusive [6] , and some are likely to be found among the numerous uncharacterized Class I MTases. Valosin-containing protein (VCP) is an abundant, essential and highly conserved AAA+ protein ( A TPase a ssociated with various cellular a ctivities) found in all eukaryotes [7] . It contains two ATPase domains, denoted D1 and D2, which form two stacked rings around a central pore in the homohexameric quaternary structure [8] . VCP is involved in a wide range of biological processes, such as cell cycle regulation, membrane fusion, autophagy and ubiquitin-mediated protein degradation, which may be explained by its ability to act as an adenosine triphosphate (ATP)-dependent chaperone [7] , [9] . Certain mutations that only modestly affect the biochemical activity of VCP cause the severe autosomal dominant disorder Inclusion body myopathy with early-onset Paget disease and/or frontotemporal dementia [10] , underscoring the importance of fine-tuning of VCP function in humans. Here we show that the putative human Class I MTase METTL21D specifically catalyses the trimethylation of Lys315 in VCP in vitro , and the enzyme was thus named VCP-lysine methyltransferase (VCP-KMT). Moreover, this previously unknown VCP modification is present in mouse tissues and human cell lines, and was abolished in the latter by zinc-finger nuclease-mediated VCP-KMT disruption. VCP-KMT was in a recent study found to be a promoter of tumour metastasis [11] , and accordingly, VCP-KMT-deficient cells showed reduced proliferation, migration and invasive potential. Finally, a combination of biochemical and bioinformatics analyses indicates that VCP-KMT belongs to a novel human protein MTase family with ten members, of which the majority seems to be lysine-specific. Bioinformatics analysis of METTL21D During our efforts to define the function of the putative human macromolecular demethylase ALKBH6, we identified the putative Class I MTase METTL21D as a potential binding partner in a yeast two-hybrid screen (S.K., E.D., P.Ø.F., unpublished observation). Although ALKBH6 was not confirmed as an interaction partner of METTL21D in a reciprocal yeast two-hybrid screen or pull-down experiments, we undertook a functional characterization of this MTase. Human METTL21D belongs to a small subfamily of four highly homologous (30–50% sequence identity) uncharacterized putative MTases, designated METTL21A-METTL21D. To identify orthologs of METTL21D, we used BLAST searches to detect proteins that were highly such as METTL21D, but showed a substantially lower similarity to METTL21A, METTL21B and METTL21C. Plausible orthologs of METTL21D are found in a wide range of multicellular eukaryotes, but show a rather scattered distribution. Vertebrates, plants, nematodes and green algae all have a METTL21D ortholog, whereas such proteins are absent in the majority of fungi and insects, such as the model organisms Saccharomyces cerevisiae and Drosophila melanogaster . Class I MTases contain a Rossmann-fold-like bundle of seven β-strands and display four characteristic conserved sequence motifs denoted I, Post I, II and III [12] . A sequence alignment of putative METTL21D orthologs indicates the presence of the characteristic core motifs, and secondary structure prediction further indicates a topology of an archetypical Class I MTase core domain with an added N-terminal elongation harbouring three short β-strands ( Fig. 1a ). This initial bioinformatics analysis consolidates METTL21D as a member of the seven β-strand MTase family, and indicates that this enzyme is present in a wide range of multicellular eukaryotes. 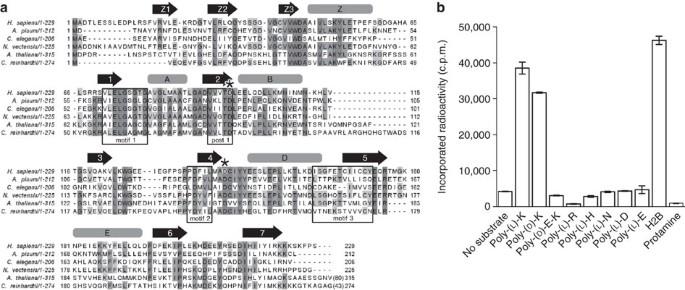Figure 1: METTL21D is a lysine-specific class I MTase. (a) Alignment of METTL21D protein sequences (H. sapiens, NP_078834;A. pisum, XP_001945214.1;C. elegans, NP_001122759.1;N. vectensis, XP_001636505.1;Arabidopsis thaliana, NP_973791.1;Chlamydomonas reinhardtii, XP_001692568.1). Predicted α-helices and β-strands of human METTL21D are indicated. Hallmark motifs are boxed. Key residues Asp96 and Asp144 are indicated by asterisks. (b) METTL21D methylates lysine-containing, positively charged model substrates. Data are represented as means ±s.d.,n=3. Figure 1: METTL21D is a lysine-specific class I MTase. ( a ) Alignment of METTL21D protein sequences ( H. sapiens , NP_078834; A. pisum , XP_001945214.1; C. elegans , NP_001122759.1; N. vectensis , XP_001636505.1; Arabidopsis thaliana , NP_973791.1; Chlamydomonas reinhardtii , XP_001692568.1). Predicted α-helices and β-strands of human METTL21D are indicated. Hallmark motifs are boxed. Key residues Asp96 and Asp144 are indicated by asterisks. ( b ) METTL21D methylates lysine-containing, positively charged model substrates. Data are represented as means ±s.d., n =3. Full size image Protein MTase activity of METTL21D When testing recombinant METTL21D for MTase activity, we were unable to detect any activity on DNA or RNA, but METTL21D displayed activity on recombinant histone proteins, for example on H2B, the most lysine-rich core histone ( Fig. 1b ). To further analyse the protein MTase activity of METTL21D, we tested homopolymers of the L -amino acids lysine (K), arginine (R), histidine (H), asparagine (N), aspartate (D) and glutamate (E), which have all been shown to be methylated in proteins [1] . Notably, METTL21D displayed MTase activity on poly-( L )-K, but not on any of the other homopolymers ( Fig. 1b ). Protein MTase activity was also observed on a homopolymer of the D -stereoisomer of lysine (not naturally found in proteins), but not on a randomized copolymer of D -glutamate and D -lysine at a ratio of 3:2 (poly-( D )-E-K). No activity could be detected on protamine, which, similar to H2B, is a highly positively charged chromatin protein, but contains no lysine. Mass spectrometry (MS) analysis of histone H2B after incubation with METTL21D and SAM identified several methylated lysine residues (not shown). From the above experiments, we concluded that METTL21D is a lysine-specific protein MTase, but that the observed modification of multiple lysine residues within H2B indicates a lack of sequence selectivity. METTL21D interacts with and methylates VCP in vitro To identify potential substrates of METTL21D, a yeast two-hybrid screen was commissioned (Hybrigenics, Paris, France), using human METTL21D as bait with a human placenta cDNA prey library. Interestingly, the majority of the interacting clones (111 of 169) encoded VCP, a much-studied protein, which belongs to the family of AAA+ proteins. These clones comprised 34 unique sequences, and shared the region encoding residues 282–364, thereby defining the so-called selected interaction domain, as being responsible for the interaction ( Fig. 2a,b ). 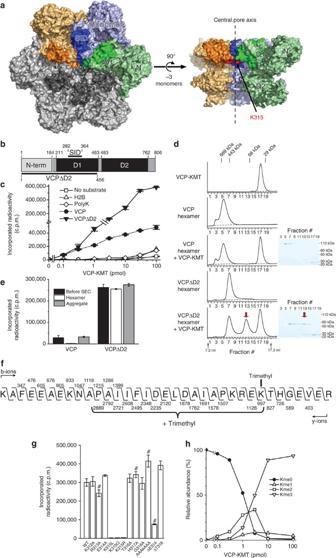Figure 2: VCP-KMT interacts with and methylates VCPin vitro. (a) Structure of hexameric VCP. Three of the protomers have been individually colour-labeled and darker colour indicates the selected interaction domain (SID) involved in VCP-KMT interaction. The structure was rendered using symmetry expansion on a published VCP structure (pdb 1oz4)8. (b) Domain structure of VCP showing the N-terminal, D1 ATPase and D2 ATPase domains, and indicating the SID and VCPΔD2. (c) VCP-KMT methylates VCP and VCPΔD2. Ten microgram of substrate were incubated with varying amounts of VCP-KMT at pH 7.5. Data are represented as means±s.d.,n=3. (d) VCP-KMT disrupts the hexamer and forms a complex with VCPΔD2. Hexameric VCP or VCPΔD2 were incubated with a twofold molar excess of VCP-KMT, followed by SEC. Left, Elution profiles (absorbance at 280 nm) of protein samples and size standards. Right, Coomassie blue-stained SDS–PAGE of indicated fractions. (e) Methylation assay using purified hexameric VCP and VCPΔD2. Ten microgram of protein before SEC, hexameric protein purified as shown in (d), or aggregated protein eluting in the void volume were incubated with 100 pmol VCP-KMT. Error bars indicate range between duplicate samples. (f) MS/MS sequencing of Arg-C generated peptide VCPΔD2(288–322)-Kme3 ([M+1H]+=4,007.124 Da) showing trimethylation of Lys315. The corresponding spectrum is shown inSupplementary Fig. S2a. (g) Mutational analysis of VCPΔD2 methylation. VCPΔD2 variants with point mutations in the region surrounding Lys315 were incubated with 100 pmol VCP-KMT. Data are represented as means±s.e.m.,n=4. Four variants (#) showed changed assembly and/or aggregation, seeSupplementary Fig. S4. (h) Methylation status of VCPΔD2 incubated with varying amounts of VCP-KMT. The methylation status of Lys315 in peptide VCPΔD2(288–322) was quantified by MS. See alsoSupplementary Fig. S2c. Figure 2: VCP-KMT interacts with and methylates VCP in vitro . ( a ) Structure of hexameric VCP. Three of the protomers have been individually colour-labeled and darker colour indicates the selected interaction domain (SID) involved in VCP-KMT interaction. The structure was rendered using symmetry expansion on a published VCP structure (pdb 1oz4) [8] . ( b ) Domain structure of VCP showing the N-terminal, D1 ATPase and D2 ATPase domains, and indicating the SID and VCPΔD2. ( c ) VCP-KMT methylates VCP and VCPΔD2. Ten microgram of substrate were incubated with varying amounts of VCP-KMT at pH 7.5. Data are represented as means±s.d., n =3. ( d ) VCP-KMT disrupts the hexamer and forms a complex with VCPΔD2. Hexameric VCP or VCPΔD2 were incubated with a twofold molar excess of VCP-KMT, followed by SEC. Left, Elution profiles (absorbance at 280 nm) of protein samples and size standards. Right, Coomassie blue-stained SDS–PAGE of indicated fractions. ( e ) Methylation assay using purified hexameric VCP and VCPΔD2. Ten microgram of protein before SEC, hexameric protein purified as shown in ( d ), or aggregated protein eluting in the void volume were incubated with 100 pmol VCP-KMT. Error bars indicate range between duplicate samples. ( f ) MS/MS sequencing of Arg-C generated peptide VCPΔD2(288–322)-Kme3 ([M+1H] + =4,007.124 Da) showing trimethylation of Lys315. The corresponding spectrum is shown in Supplementary Fig. S2a . ( g ) Mutational analysis of VCPΔD2 methylation. VCPΔD2 variants with point mutations in the region surrounding Lys315 were incubated with 100 pmol VCP-KMT. Data are represented as means±s.e.m., n =4. Four variants (#) showed changed assembly and/or aggregation, see Supplementary Fig. S4 . ( h ) Methylation status of VCPΔD2 incubated with varying amounts of VCP-KMT. The methylation status of Lys315 in peptide VCPΔD2(288–322) was quantified by MS. See also Supplementary Fig. S2c . Full size image We then tested whether VCP is a substrate for recombinant METTL21D in an MTase assay. The selected interaction domain is located in the D1 ATPase domain and appears inaccessible in the VCP hexamer structure; therefore, a VCP deletion mutant (VCPΔD2) that lacks the D2 ATPase domain ( Fig. 2b ) and forms a less stable hexamer [13] , [14] was also tested. Indeed, both VCP and VCPΔD2 were methylated by METTL21D in vitro , but considerably higher levels of methylation were obtained in the case of VCPΔD2 ( Fig. 2c ). Notably, the activity on VCP/VCPΔD2 was much stronger than that on histone H2B and poly-( L )-lysine; the METTL21D concentration required to detect activity was ~300-fold lower and the obtained methylation levels up to ~40-fold higher. On the basis of the robust activity of METTL21D on VCP, we henceforth denote this enzyme as VCP-KMT. The observation that VCPΔD2 was a considerably better substrate than VCP suggested that VCP-KMT might be able to disrupt the hexameric structure of VCPΔD2 to exert its MTase activity, and that this could only occur efficiently with the less stable VCPΔD2 mutant. Indeed, incubation of the ~300 kDa homohexameric VCPΔD2 complex with VCP-KMT led to the formation of heterodimeric VCP-KMT:VCPΔD2 that eluted at ~80 kDa in size exclusion chromatography (SEC) ( Fig. 2d ) and the purified hexameric VCPΔD2 was an efficient substrate for VCP-KMT ( Fig. 2e ). The more stable full-length VCP hexamer was not disrupted by VCP-KMT ( Fig. 2d ), and although aggregated VCP contained in the VCP preparation could be methylated, no methylation of intact hexameric VCP was observed ( Fig. 2e ). In addition, no in vitro methylation of endogenous VCP in a cytosolic fraction from wild-type and VCP-KMT-deficient HeLa cells was detected ( Supplementary Fig. S1 ). This suggests that VCP-KMT-mediated methylation of VCP occurs before hexamer assembly in vivo . VCP-KMT methylates lysine 315 of VCP To identify the site(s) of VCP-KMT-mediated methylation in VCP, in vitro methylated VCPΔD2 was analysed by MS. Among peptides covering 88% of VCPΔD2, a single lysine residue, Lys315, was found to be trimethylated in the VCP-KMT-treated sample, but not in the untreated control sample, and no other methylated residues were detected ( Fig. 2f ; Supplementary Fig. S2a ). In agreement with these data, the VCP mutant K315L was not subject to VCP-KMT-mediated methylation ( Fig. 2g ; Supplementary Fig. S2b ), strongly indicating that Lys315 is the only methylation site. Substrate and enzyme requirements for VCP-KMT activity Protein lysine MTases recognize their substrates either through interaction with a short linear target sequence or by binding to a more complex three-dimensional structure. To elucidate the mode of substrate recognition for VCP-KMT, we tested its activity on various VCP-derived substrates. No methylation was observed on glutathione S -transferase fusions of two short (13 and 21 aa) peptides representing the methylation site and surrounding residues, regardless of whether the peptides were liberated from glutathione S -transferase by site-specific proteolytic cleavage ( Supplementary Fig. S3 ). This indicates that a larger portion of VCP is required for productive interaction with VCP-KMT. When three residues at either side of the methylation site in VCPΔD2 were individually replaced by alanine, none of the six mutations affected VCP-KMT-mediated methylation, nor did a simultaneous replacement of all six residues ( Fig. 2g ). However, a deletion of the amino acid N-proximal to the methylation site (ΔE314) caused aberrant oligomerization and a fourfold reduction in methylation, whereas a corresponding C-proximal deletion (ΔT316) had no effect ( Fig. 2g ; Supplementary Fig. S4 ). In addition to lysine, other large polar residues can be N-methylated, and we considered the possibility that such amino acids may be methylated by VCP-KMT when placed in an appropriate structural context. We therefore mutated Lys315 of VCPΔD2 into Arg or Gln, but similar to the K315L variant, these mutants were not methylated ( Fig. 2g ) although they efficiently formed hexamers ( Supplementary Fig. S4 ). In conclusion, our data indicate that VCP-KMT specifically recognizes and methylates a lysine residue placed in a given three-dimensional context, whereas the local sequence surrounding the methylation site is less important for recognition. To examine the processivity of the methylation reaction, VCPΔD2 was incubated with different amounts of VCP-KMT and the methylation status of Lys315 was analysed by MS ( Fig. 2h and Supplementary Fig. S2c ). Although nearly all VCP was trimethylated at high VCP-KMT concentrations, we observed a mixture of all four lysine methylation states (Kme0, Kme1, Kme2 and Kme3) at intermediate concentrations. This suggests a non-processive reaction mechanism as has been described for DOT1 [15] . Finally, we analysed mutants of VCP-KMT to pinpoint residues critical to MTase activity ( Supplementary Fig. S5 ). A conserved Asp residue in motif Post I is among the most conserved residues in Class I MTases [16] and has been shown to have an important role in coordinating SAM [17] . Accordingly, mutations at this position in VCP-KMT (D96A, D96V) almost completely abolished enzymatic activity. Furthermore, the mutation D144V, which disrupts the (D/E)-X-X-(Y/F) motif present in VCP-KMT and its nine closest homologs (see below and Fig. 6a), also abolished methylation activity. VCP-KMT-mediated trimethylation of Lys315 in VCP in vivo We observed highly efficient and specific VCP-KMT-mediated methylation of Lys315 in VCP in vitro , suggesting that the corresponding methylation may also occur in vivo . To address this, we isolated VCP by immunoprecipitation from protein extracts from mouse brain, heart, kidney, liver and testicle, and investigated the methylation status of Lys315 by MS analysis. In all five tissues, VCP was almost completely trimethylated, with only trace amounts of the dimethylated form present ( Fig. 3a ). 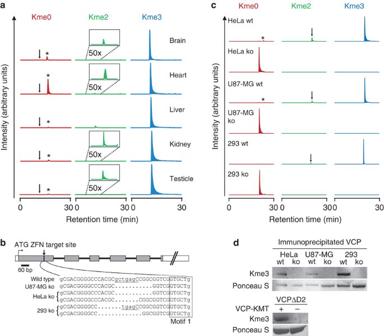Figure 3: VCP-KMT-mediated trimethylation of VCPin vivo. (a) MS-analysis of VCP isolated from mouse tissues. Chromatograms for un-, di- and trimethylated Lys315 in Arg-C-generated peptide VCP(314–322) are shown. Selective ion settings were m/z=542.7727, 556.7884 and 563.7962±6 p.p.m.,z=+2. For each tissue, the intensity is normalized to the Kme3 signal. Expected elution time of the Kme0 peptide (arrows) and irrelevant peaks (*, M+1 isotope peak of an unrelated peptide) are indicated. Monomethylated peptide was not detected. (b) Zinc-finger nuclease-mediated disruption of theVCP-KMTgene in human cell lines. In a schematic representation of the humanVCP-KMTgene, boxes indicate the coding (grey) and non-coding (light grey) parts of exons, whereas solid black lines indicate introns (not to scale). A blow-up of the sequence at the ZFN target site is shown. ZFN cleavage is expected to occur between the two ZFN-binding sites (uppercase). The genotypes of selected clones harbouring frame shift mutations are shown. U87-MG cells contain only a single copy of theVCP-KMTgene. (c) MS-analysis of VCP isolated from wild-type and VCP-KMT-deficient cell lines. Settings as in (a). For each cell line, the chromatograms are normalized to the highest intensity measured. Kme2 peptides (arrows) and irrelevant peaks (*, M+1 isotope peak of an unrelated peptide) are indicated. (d) Assessment of VCP methylation by western blot. Upper panel, western blot of immunoprecipitated VCP from wild-type and VCP-KMT-deficient cell lines using pan-Kme3 antibody. Lower panel, similar blot ofin vitromethylated VCPΔD2 (positive control). A Ponceau S stain of the membrane is shown as loading control. Figure 3: VCP-KMT-mediated trimethylation of VCP in vivo . ( a ) MS-analysis of VCP isolated from mouse tissues. Chromatograms for un-, di- and trimethylated Lys315 in Arg-C-generated peptide VCP(314–322) are shown. Selective ion settings were m/z=542.7727, 556.7884 and 563.7962±6 p.p.m., z =+2. For each tissue, the intensity is normalized to the Kme3 signal. Expected elution time of the Kme0 peptide (arrows) and irrelevant peaks (*, M+1 isotope peak of an unrelated peptide) are indicated. Monomethylated peptide was not detected. ( b ) Zinc-finger nuclease-mediated disruption of the VCP-KMT gene in human cell lines. In a schematic representation of the human VCP-KMT gene, boxes indicate the coding (grey) and non-coding (light grey) parts of exons, whereas solid black lines indicate introns (not to scale). A blow-up of the sequence at the ZFN target site is shown. ZFN cleavage is expected to occur between the two ZFN-binding sites (uppercase). The genotypes of selected clones harbouring frame shift mutations are shown. U87-MG cells contain only a single copy of the VCP-KMT gene. ( c ) MS-analysis of VCP isolated from wild-type and VCP-KMT-deficient cell lines. Settings as in ( a ). For each cell line, the chromatograms are normalized to the highest intensity measured. Kme2 peptides (arrows) and irrelevant peaks (*, M+1 isotope peak of an unrelated peptide) are indicated. ( d ) Assessment of VCP methylation by western blot. Upper panel, western blot of immunoprecipitated VCP from wild-type and VCP-KMT-deficient cell lines using pan-Kme3 antibody. Lower panel, similar blot of in vitro methylated VCPΔD2 (positive control). A Ponceau S stain of the membrane is shown as loading control. Full size image To analyse whether VCP-KMT is the enzyme responsible for VCP methylation in vivo , we disrupted the VCP-KMT gene in three different human cell lines: HeLa (epithelial), U87-MG (glioma) and 293 T-REx Flp-In (kidney). A pair of zinc-finger nucleases was designed to specifically target exon 1 of the VCP-KMT gene upstream of motif I (aa 71–79) ( Fig. 3b ). When zinc-finger nucleases cut a coding sequence, imperfect repair by non-homologous end-joining frequently leads to indel mutations, and a frameshift mutation at the targeted site in the VCP-KMT gene will lead to the loss of almost the entire MTase core domain. Clones harbouring frameshift mutations in all VCP-KMT alleles were obtained for all three cell lines ( Fig. 3b ). We next analysed the methylation status of VCP from wild-type and VCP-KMT-deficient cells. Similar to the observations from mouse tissues, VCP was almost completely trimethylated in all three wild-type cell lines, whereas no methylation was detected in VCP-KMT-deficient cells ( Fig. 3c ). Immunoprecipitation of VCP followed by western blotting with pan-Kme3 antibody further confirmed the methylation status of Lys315 and the absence of other trimethylated lysines ( Fig. 3d ). Taken together, these results show that VCP is almost completely trimethylated at position Lys315 in a variety of mammalian cell lines and tissues, and that VCP-KMT is the responsible enzyme. Organismal distribution of VCP methylation VCP appears to be present in all eukaryotes, whereas VCP-KMT shows a far more limited distribution. For example, the yeast S. cerevisiae has an apparent homologue of the METTL21 proteins (YNL024c), but this protein is more similar to METTL21A than to VCP-KMT. Indeed, recombinant YNL024c failed to show MTase activity on human VCPΔD2 or on the corresponding yeast protein CDC48ΔD2, whereas human VCP-KMT was active on both these substrates ( Fig. 4a ). Moreover, the peptide containing Lys325 (corresponding to Lys315 in human VCP) was exclusively found in a non-methylated state in CDC48 isolated from yeast cells ( Fig. 4b ). To address whether a putative VCP-KMT ortholog from an organism distantly related to humans also displayed VCP-specific MTase activity, we investigated protein C42C1.13 from the nematode Caenorhabditis elegans . Indeed, this protein showed even higher activity than human VCP-KMT on both human VCPΔD2 and yeast CDC48ΔD2 ( Fig. 4c ). Taken together, the absence of VCP methylation in S. cerevisiae and the observed activity of the C. elegans protein C42C1.13 on both yeast and human VCP indicate that VCP-methylation can occur in a wide range of eukaryotes but is absent in those that lack a VCP-KMT ortholog. 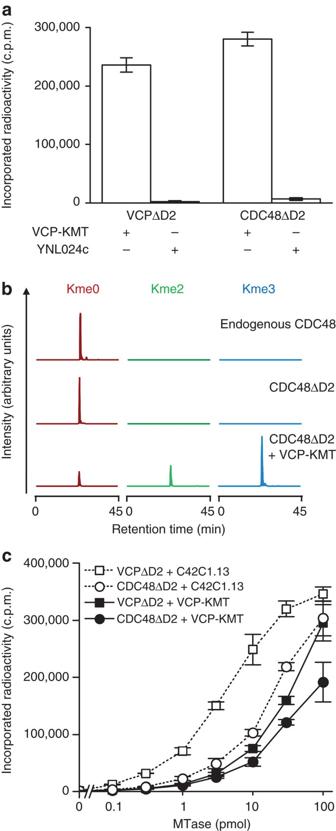Figure 4: VCP methylation in other organisms. (a) Lack of VCP-specific MTase activity ofS. cerevisiaeYNL024c. VCPΔD2 and the orthologous yeast protein CDC48ΔD2 were incubated with 100 pmol VCP-KMT or YNL024c. (b) Lack of CDC48 methylation inS. cerevisiae. Chromatograms representing different K325 methylation states for chymotryptic peptide CDC48(313–338) are shown. Selective ion settings were m/z=742.9026, 749.9104 and 753.4144±10 p.p.m.,z=+4. Top, CDC48 isolated fromS. cerevisiae. Middle, untreated recombinant CDC48ΔD2 (negative control). Bottom, VCP-KMT-treated CDC48ΔD2 (positive control for detection of methylated peptides). (c) VCP-KMT activity ofC. elegansprotein C42C1.13. Human VCPΔD2 and yeast CDC48ΔD2 were incubated with varying amounts of C42C1.13 or human VCP-KMT. Data in (a,c) are represented as means ±s.d.,n=3. Figure 4: VCP methylation in other organisms. ( a ) Lack of VCP-specific MTase activity of S. cerevisiae YNL024c. VCPΔD2 and the orthologous yeast protein CDC48ΔD2 were incubated with 100 pmol VCP-KMT or YNL024c. ( b ) Lack of CDC48 methylation in S. cerevisiae . Chromatograms representing different K325 methylation states for chymotryptic peptide CDC48(313–338) are shown. Selective ion settings were m/z=742.9026, 749.9104 and 753.4144±10 p.p.m., z =+4. Top, CDC48 isolated from S. cerevisiae . Middle, untreated recombinant CDC48ΔD2 (negative control). Bottom, VCP-KMT-treated CDC48ΔD2 (positive control for detection of methylated peptides). ( c ) VCP-KMT activity of C. elegans protein C42C1.13. Human VCPΔD2 and yeast CDC48ΔD2 were incubated with varying amounts of C42C1.13 or human VCP-KMT. Data in ( a , c ) are represented as means ±s.d., n =3. Full size image Functional importance of VCP methylation As VCP was non-methylated in VCP-KMT-deficient cells, we used these cells to address the biological significance of VCP methylation. No appreciable difference between VCP-KMT-proficient and -deficient cells was detected in degradation assays using reporters of the ubiquitin proteasome system or when monitoring autophagy by LC3B processing ( Supplementary Figs S6,S7 ). We were intrigued by a very recent study reporting that VCP-KMT, there denoted NVM-1, was upregulated in a number of metastatic tumours, and that it was required for efficient cell migration and invasion [11] . First, we performed proliferation assays where the various VCP-KMT-deficient cell lines were compared with their wild-type counterparts. These experiments showed a significantly increased doubling time for VCP-KMT-deficient HeLa and 293 T-REx Flp-In cells, but not for the slower growing U87-MG cells ( Fig. 5a,b ). 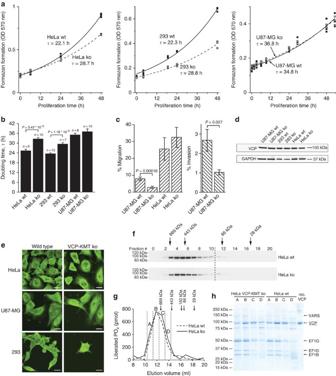Figure 5: Effects ofVCP-KMTdisruption on cellular phenotypes and VCP function. (a) Representative growth curves of HeLa (left), 293 T-REx Flp-In (middle) and U87-MG cells (right). An exponential fit to the data is shown and the deduced doubling timeôis indicated. (b) Doubling time of wild-type and VCP-KMT-deficient cell lines. Data are represented as means±s.e.m.,nis indicated. Significant differences between means are indicated (alpha level 0.05, two-tailed independent two-sample Student'st-test) andP-values are shown. (c) Migration and invasion of wild-type and VCP-KMT-deficient cells. HeLa and U87-MG cells were assayed in a transwell assay with or without Matrigel coating. The percentage of cells having traversed the filter after 24 h is shown. Data are represented as means±s.e.m.,n=4. Significant differences between means are indicated (alpha level 0.05, two-tailed independent two-sample Student'st-test) andP-values are shown. (d) VCP content of wild-type and VCP-KMT-deficient cell lines. Whole-cell lysate (7.5 μg protein) was separated by SDS–PAGE and subjected to western blot with VCP- and glyceraldehyde-3-phosphate dehydrogenase (GAPDH)-specific antibodies. (e) Localization of VCP in wild-type and VCP-KMT-deficient cells. Fixed and permeabilized cells were stained with VCP-specific antibody. Az-projection of a stack of confocal images is shown. Scale bar=20 μm. (f) Size of endogenous VCP complexes. S100 fractions from HeLa wt and VCP-KMT-deficient cells were separated by SEC and fractions were analysed by anti-VCP western blot. (g) ATPase activity of VCP from wild-type and VCP-KMT-deficient cells. VCP was partially purified from wild-type or VCP-KMT-deficient HeLa cells by anion exchange chromatography and SEC, and the ATPase activity of SEC fractions was measured. (h) Coomassie-stained SDS–PAGE of VCP-containing SEC fractions A–D. Copurified Valyl-tRNA synthetase complex subunits and VCP were identified by MS (arrows). Figure 5: Effects of VCP-KMT disruption on cellular phenotypes and VCP function. ( a ) Representative growth curves of HeLa (left), 293 T-REx Flp-In (middle) and U87-MG cells (right). An exponential fit to the data is shown and the deduced doubling time ô is indicated. ( b ) Doubling time of wild-type and VCP-KMT-deficient cell lines. Data are represented as means±s.e.m., n is indicated. Significant differences between means are indicated (alpha level 0.05, two-tailed independent two-sample Student's t -test) and P -values are shown. ( c ) Migration and invasion of wild-type and VCP-KMT-deficient cells. HeLa and U87-MG cells were assayed in a transwell assay with or without Matrigel coating. The percentage of cells having traversed the filter after 24 h is shown. Data are represented as means±s.e.m., n =4. Significant differences between means are indicated (alpha level 0.05, two-tailed independent two-sample Student's t -test) and P -values are shown. ( d ) VCP content of wild-type and VCP-KMT-deficient cell lines. Whole-cell lysate (7.5 μg protein) was separated by SDS–PAGE and subjected to western blot with VCP- and glyceraldehyde-3-phosphate dehydrogenase (GAPDH)-specific antibodies. ( e ) Localization of VCP in wild-type and VCP-KMT-deficient cells. Fixed and permeabilized cells were stained with VCP-specific antibody. A z -projection of a stack of confocal images is shown. Scale bar=20 μm. ( f ) Size of endogenous VCP complexes. S100 fractions from HeLa wt and VCP-KMT-deficient cells were separated by SEC and fractions were analysed by anti-VCP western blot. ( g ) ATPase activity of VCP from wild-type and VCP-KMT-deficient cells. VCP was partially purified from wild-type or VCP-KMT-deficient HeLa cells by anion exchange chromatography and SEC, and the ATPase activity of SEC fractions was measured. ( h ) Coomassie-stained SDS–PAGE of VCP-containing SEC fractions A–D. Copurified Valyl-tRNA synthetase complex subunits and VCP were identified by MS (arrows). Full size image We also examined whether the VCP-KMT-deficient cells may have reduced migratory or invasive capacity. A Boyden Chamber assay with uncoated and matrigel-coated membranes allowed us to distinguish between migration and invasion, respectively ( Fig. 5c ). Wild-type U87-MG cells showed significantly higher migration and invasion potential than VCP-KMT-deficient U87-MG cells. Wild-type and VCP-KMT-deficient HeLa cells showed similar migratory capacity ( Fig. 5c ) and no invasive potential. 293 T-REx Flp-In cells were not analysed due to their limited migration capability. The growth-related differences between wild-type and VCP-KMT-deficient cells could conceivably be caused by changes in the stability or biochemical properties of VCP. Therefore, we first examined the amount, complex size and subcellular distribution of VCP by western blotting and immunofluorescence staining, but we did not detect any differences between wild-type and VCP-KMT-deficient cells ( Fig. 5d-f ). Furthermore, we investigated the possible effect of methylation on the ATPase activity of VCP ( Fig. 5g ). To this end, we used anion exchange chromatography followed by SEC to isolate VCP-complexes from HeLa cells. VCP was the predominant protein in the complex-containing fractions, but a copurifying complex consisting of the Valyl-tRNA synthetase (VARS) and the β, γ and δ subunits of translation elongation factor 1 (EF1) [18] was also detected ( Fig. 5h ). The complex-containing fractions displayed an expected ATPase activity, which showed an elution profile similar to that of VCP, whereas the VARS/EF1 complex eluted somewhat earlier, indicating that the measured activity primarily is due to VCP. However, no appreciable difference in ATPase activity of samples from VCP-KMT-proficient and -deficient HeLa cells was detected, indicating that methylation does not substantially influence the basal ATPase activity of VCP in vitro . VCP-KMT belongs to a family of novel protein MTases VCP-KMT belongs to Family 16 of MTases (InterPro: IPR019410; Pfam: PF10294), which has ten human members, and we performed a more detailed bioinformatics analysis of this MTase family. The ten human members form a closed group of proteins that invariably retrieve each other as best hits in BLAST searches, and orthologs of most of these proteins are found in a wide range of eukaryotic species ( Table 1 ). Interestingly, one of these proteins, C2orf34, was recently shown to be the long-sought MTase responsible for trimethylation of Lys115 in calmodulin (CaM-KMT) [4] , whereas YIL110W, the closest yeast homolog of human Family 16 member C1orf156, was recently shown to be required for monomethylation of the ribosomal protein Rpl3 on His243 [19] . Notably, CaM-KMT and C1orf156 are among the human Family 16 proteins that display the lowest sequence similarity to VCP-KMT ( Table 1 ). Table 1 Human family 16 MTases and their putative orthologs. Full size table VCP-KMT orthologs contain a conserved DXXY motif located immediately C-terminal to Motif II ( Fig. 1a ). A more general expansion of this motif, (D/E)XX(Y/F), is present in all ten human Family 16 members ( Fig. 6a ), and in their orthologs from other organisms (not shown). A similar, so-called DPPY motif, with consensus (D/N/S)PP(Y/F), is found at the corresponding position in DNA N 6 -adenine MTases, DNA N 4 -cytosine MTases and the protein glutamine MTase HemK [20] . Here, the first residue has an important role in methyl transfer, and mutation at this position leads to a catalytically inactive enzyme. We observed that mutation of the corresponding residue Asp144 in VCP-KMT inactivated the enzyme ( Supplementary Fig. S5 ), suggesting that the (D/E)XX(Y/F) motif in the Family 16 proteins may have a similar role as the DPPY motif. 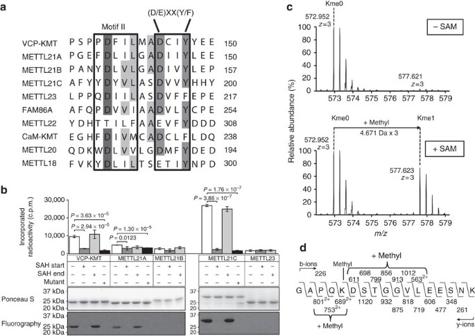Figure 6: Protein MTase activity of additional human Family 16 proteins. (a) Sequence alignment of the ten human Family 16 proteins showing the hallmark (D/E)XX(Y/F) motif located downstream of Motif II. (b) Automethylation activity of selected MTase Family 16 members. 300 pmol of MT were incubated for 1 h at pH 8.5 with [3H]-SAM. The competitive inhibitorS-adenosyl homocysteine (SAH) was added at the start or end of the incubation to distinguish between automethylation and SAM-binding. Top, liquid scintillation counting results, data are represented as means±s.d.,n=3. Significant effects of mutation or SAH addition on mean incorporated radioactivity are indicated (alpha level 0.05, one-tailed independent two-sample Student'st-test) andP-values are shown. Bottom, Ponceau S staining and fluorography of duplicate samples separated by SDS–PAGE and blotted on polyvinylidene difluoride (PVDF) membrane. (c) Lysine-specific automethylation of METTL21C. A mass shift corresponding to monomethylation of tryptic peptide METTL21C(31–47) is detected upon incubation of METTL21C with SAM. (d) MS/MS sequencing of peptide METTL21C(31–47)-Kme1 ([M+1H]+1,730.856 Da) showing lysine monomethylation on residue Lys35. The masses of detected b- and y-ions are indicated. The corresponding spectrum is shown inSupplementary Fig. S8. Figure 6: Protein MTase activity of additional human Family 16 proteins. ( a ) Sequence alignment of the ten human Family 16 proteins showing the hallmark (D/E)XX(Y/F) motif located downstream of Motif II. ( b ) Automethylation activity of selected MTase Family 16 members. 300 pmol of MT were incubated for 1 h at pH 8.5 with [ 3 H]-SAM. The competitive inhibitor S -adenosyl homocysteine (SAH) was added at the start or end of the incubation to distinguish between automethylation and SAM-binding. Top, liquid scintillation counting results, data are represented as means±s.d., n =3. Significant effects of mutation or SAH addition on mean incorporated radioactivity are indicated (alpha level 0.05, one-tailed independent two-sample Student's t -test) and P -values are shown. Bottom, Ponceau S staining and fluorography of duplicate samples separated by SDS–PAGE and blotted on polyvinylidene difluoride (PVDF) membrane. ( c ) Lysine-specific automethylation of METTL21C. A mass shift corresponding to monomethylation of tryptic peptide METTL21C(31–47) is detected upon incubation of METTL21C with SAM. ( d ) MS/MS sequencing of peptide METTL21C(31–47)-Kme1 ([M+1H] + 1,730.856 Da) showing lysine monomethylation on residue Lys35. The masses of detected b- and y-ions are indicated. The corresponding spectrum is shown in Supplementary Fig. S8 . Full size image Five out of the ten human Family 16 proteins, VCP-KMT, METTL21A, METTL21B, METTL21C and METTL23, form the distinct subfamily PTHR14614 in the PANTHER database [21] . To address whether these closest paralogs of VCP-KMT are also protein MTases, in vitro methylation experiments were performed. Unlike VCP-KMT, METTL21A–C and METTL23 failed to show MTase activity towards histones, amino-acid homopolymers or VCP. Some protein MTases display automethylation activity, and then with an amino-acid specificity identical to that observed for bona fide substrates [22] , [23] , [24] . Indeed, we detected significant automethylation in the case of METTL21A, METTL21C and VCP-KMT ( Fig. 6b ). The observed automethylation activity was sensitive to the competitive inhibitor S -adenosyl homocysteine when added at the beginning, but not at the end of the incubation period, indicating that the observed activity reflects bona fide methylation, rather than non-covalent association of [ 3 H]-SAM with the enzymes' SAM-binding sites. The automethylation activity of VCP-KMT, METTL21A and METTL21C was abrogated by mutations (D96A, D94A and D141A, respectively) of the conserved SAM-binding Asp residue in Motif Post 1, which in the case of VCP-KMT abrogated VCP methylation. The level of automethylation was particularly high in the case of METTL21C, where substantial (~50%) monomethylation at a specific lysine residue, Lys35, was detected by MS ( Fig. 6c,d and Supplementary Fig. S8 ). Our observed protein MTase activity of METTL21A, METTL21C and VCP-KMT, taken together with CaM-KMT and C1orf156 already being implicated in protein methylation, clearly suggests that all ten human Family 16 members are protein MTases. The majority of lysine-specific protein MTases (KMTs) belong to the SET-domain family, and until now, only two human Class I KMTs have been described, namely CaM-KMT and DOT1L. Here, by using both in vitro and in vivo strategies, we firmly establish the existence of a third such enzyme, VCP-KMT, which is responsible for the trimethylation of VCP on Lys315. In a recent study, 119 genes that were upregulated in a metastatic cancer cell line were subjected to secondary screens, pin-pointing a single gene, denoted NVM-1 (novel metastasis-promoting gene 1), as being particularly important for migratory behaviour and metastatic potential [11] . Interestingly, NVM-1 is identical to VCP-KMT. In the present study, we found that genetic ablation of VCP-KMT in human cell lines affected cell growth, migration and invasion, further supporting the notion that VCP-KMT is important for cancer metastasis. VCP-KMT expression may promote cancer cell migration and metastasis by two alternative mechanisms. Conceivably, high expression of VCP-KMT in rapidly growing cancer cells might ensure optimal VCP function through efficient methylation of newly synthesized VCP. Indeed, elevated VCP expression leads to increased cell proliferation and is correlated with metastasis and cancer [25] . Alternatively, high expression of VCP-KMT may drive cancer metastasis through methylation of proteins other than VCP, that is through the methylation of a yet unidentified bona fide substrate, or through aberrant methylation of other proteins. Finally, the formal possibility exists that increased metastasis is mediated by a yet unidentified, methylation-independent function of VCP-KMT. In an effort to identify additional substrates, we used VCP-containing cytosolic S100 fraction from VCP-KMT-deficient cells ( Supplementary Fig. S1 ), or a protein macroarray containing over 3,500 denatured proteins including VCP (UniPEx_2, RZPD, Germany), as in vitro substrates. No new VCP-KMT substrates could be detected in these experiments; even VCP, although present in both assays, was not identified. Our inability to detect VCP methylation in these experiments is not unexpected, as VCP-KMT is inactive on the intact VCP hexamer (substrate in S100 assay), and requires a folded substrate (proteins immobilized on array are denatured). In line with these results, analysis of histone H3 methylation from wild-type and VCP-KMT-deficient HeLa cells by MS showed no differences in methylation. Taken together, our results indicate that the VCP-KMT activity is highly specific for VCP, although the existence of additional relevant substrates cannot be ruled out. As ALKBH6 was initially identified as a putative binding partner of VCP-KMT (S.K., E.D., P.Ø.F., unpublished observation), we tested its influence on VCP methylation in vitro . The presence of ALKBH6 did not influence the methylation activity of VCP-KMT on VCP or VCPΔD2, nor did ALKBH6 demethylate VCPΔD2 ( Supplementary Fig. S9 ). This is in line with the quantitative trimethylation of VCP seen in cell lines and mouse tissues, suggesting that reversal of VCP methylation is unlikely to occur. VCP is a highly conserved and essential protein in eukaryotes and affects many cellular processes through its central function as a molecular chaperone. In contrast, putative VCP-KMT orthologs are only found in certain eukaryotes, including vertebrates, and we found VCP to be unmethylated in the yeast S. cerevisiae , which lacks such an ortholog. Moreover, mutation at Lys315 did not strongly affect VCP function [26] . Accordingly, we found VCP-KMT-deficient human cells to be viable, showing no detectable impairment of the ubiquitin–proteasome system or autophagy, and unmethylated VCP isolated from such cells displayed ATPase activity similar to that of VCP isolated from wild-type cells. Taken together, this indicates that trimethylation at Lys315 is not required for basic VCP function, but may serve a more specialized purpose in VCP-KMT-containing organisms, supported by the observed effects of VCP-KMT knockout on cell growth and migration. VCP-KMT belongs to Family 16 of MTases, which is almost identical to what was denoted 'Group J' in a recent bioinformatics study, the major difference being that the FAM86 proteins are part of Family 16 but excluded from Group J [2] . Two out of the ten human members of this family have previously been implicated in protein methylation, CaM-KMT [4] and C1orf156 (ref. 19 ). In the present work, we have detected protein MTase activity for three human Family 16 members, namely VCP-KMT, METTL21A and METTL21C, and shown that two of these enzymes are lysine-specific. We conclude that all ten human Family 16 members are probable protein MTases, many of which are likely to be lysine-specific. Constructs and protein purification Plasmid 12373: pBD-0001, plasmid 12281: pBD-0005 (ref. 26 ) and plasmid 17229: pQE9-His-p97deltaD2 (ref. 27 ) were obtained from AddGene (URL: www.addgene.org ). Human VCP-KMT (Genbank nucleotide core accession code NM_024558.2 coding for Q9H867-4) was amplified from IMAGE:5197291. Human METTL21A (Genbank nucleotide core accession code NM_001127395.1 : 575C>T, rs2551949, coding for Q8WXB1 T192I) was cloned from HeLa cell cDNA. Human METTL21B (Genbank nucleotide core accession code NM_015433.2 : rs923829, coding for Q96AZ1) and METTL21C (Genbank nucleotide core accession code NM_001010977.1 43G>C, rs2390760, coding for Q5VZV1 G15R) were cloned from A-704 cell cDNA. The indicated single nucleotide polymorphisms represent the major alleles in the population cohorts participating in the NHLBI Exome Sequencing project. A variant of human METTL23 (Genbank nucleotide core accession code BC045819.1 with an artificial start codon introduced, coding for AAH45819 Δ1-69, L70M) was cloned from A-704 cell cDNA. C. elegans C42C1.13 (Genbank nucleotide core accession code NM_001129287.1 ) was amplified from cDNA. S. cerevisiae YNL024c (Genbank nucleotide core accession code NM_001182863.1 ) was amplified from genomic DNA of strain BY4741. VCP-KMT was cloned into MCS1 of pETDuet-1 (Novagen), other amplificates were cloned into pET28a (Novagen). Site-directed mutagenesis was performed using Quikchange II site-directed mutagenesis kit (Stratagene). Proteins were produced using standard methods [28] , [29] , variations are described in the Supplementary Methods . MTase assays MTase reactions contained 10 μg of substrate, 100 pmol MTase and 13 μM of [ 3 H]-SAM (1.5. Ci mmol −1 ) in 50 μl of 50 mM Tris–HCl, 50 mM KCl and 5 mM MgCl 2 , unless otherwise indicated. The pH value was 7.5 at 37 °C for methylation of VCP or 8.5 at 37 °C for automethylation and methylation of pseudosubstrates. After 1 h at 37 °C, the reaction was terminated by adding ice-cold 10% trichloroacetic acid followed by filtration on GF/C glass microfibre filters (Whatman). Acid-insoluble radioactivity was measured by liquid scintillation counting using Ultima Gold XR (Perkin-Elmer). For fluorography and MS analysis, reactions were stopped by adding SDS–polyacrylamide gel electrophoresis (SDS–PAGE) sample buffer and heat denaturation. For fluorography, proteins were separated by SDS–PAGE and transferred to polyvinylidene difluoride membranes, which were dried and sprayed three times with En3Hance (Perkin-Elmer). Kodak BioMax MR film was exposed to the membranes at –80 °C. For MS analysis, [ 3 H]-SAM was replaced with 1.2 mM unlabeled SAM. Analysis of VCP–VCP-KMT complex formation Recombinant monomeric VCP-KMT, hexameric VCP and hexameric VCPΔD2 were isolated by SEC in 10 mM Tris pH 8.0, 100 mM NaCl and 1 mM dithiothreitol (DTT) on a Superdex 200 10/300 GL column (GE Healthcare). Following concentration, VCP and VCPΔD2 were mixed with a twofold molar excess of VCP-KMT, incubated for 30 min at 4 °C and then rerun over the Superdex 200 column. Sample preparation, MS data acquisition and MS data analysis Protein samples to be analysed by MS were processed and analysed by nanoflow on-line liquid chromatographic MS analysis as described [30] , using either trypsin (Sigma-Aldrich), chymotrypsin (Roche Applied Science) or Arg-C (Roche Applied Science). A graphite precolumn was used for collection of the data presented in Fig. 3c . MS data were analysed with the in-house-maintained human proteome and human VCP single protein database using SEQUEST. The mass tolerances of fragment and parent ions were set to 0.05 Da and 7 p.p.m. for higher-energy collisional dissociation, and 0.5 Da and 6 p.p.m. for collision-induced dissociation, unless otherwise indicated. The following modifications were selected for analysis: methionine oxidation, Kme1, Kme2, Kme3, K-Ac, Rme1, Rme2, R-Ac, Hme1, Nme1 and Qme1 (all variable), as well as cysteine carbamidomethylation (fixed). Specific MS 2 spectra were manually inspected with Qual Browser version 2.0.7. Relative quantification of peptides with different methylation states was performed using MaxQuant [31] . Unmethylated peptide was normalized to the sample without enzyme addition and reaction products were normalized to the sum of all reaction products at the given enzyme concentration. Cell culture and generation of VCP-KMT-deficient cell lines HeLa, U87-MG and 293 T-REx Flp-In cells (Invitrogen) were cultivated in DMEM high glucose medium (Lonza) supplemented with 10% fetal bovine serum (FBS), Glutamax I (Invitrogen) and penicillin/streptomycin. The cells were transfected with mRNA encoding a zinc-finger nuclease pair targeting exon 1 of human METTL21D (Sigma-Aldrich) using Trans-IT mRNA transfection kit (Mirus BIO) and subsequently cloned by limiting dilution. Genomic DNA was prepared and a 789 bp fragment containing the ZFN target site was amplified by PCR with primers 5′-TGCTACGACTACAGCAGTATAGCTC-3′ and 5′-TGGTCCCTGGTGACTTTTATCTTC-3′. The wild-type sequence targeted by the ZFN pair constitutes a Blp I-cleavage site, enabling primary screening by Blp I-digestion of the PCR product. Uncut PCR product was sequenced to verify the genome editing and select clones with frameshift mutations. Western blotting and immunoprecipitation Adherent cells and mouse tissues were lysed in buffer containing 1% IGEPAL CA-630. A S. cerevisiae strain BY4741 cell lysate was prepared with a MicroBeadBeater. Immunoprecipitation of VCP or CDC48 was performed with antibody to VCP (ab11433, Abcam) as described [32] . For western blotting, antibody to VCP (ab11433, Abcam), rabbit polyclonal antibody to trimethylated lysine (ab76118) (Abcam) and antibody to glyceraldehyde-3-phosphate dehydrogenase (Ambion) were used according to manufacturers' suggestions. Invasion, migration and proliferation assays Cells were analysed in transwell chambers with or without matrigel coating to distinguish between invasion and migration, respectively, as described previously [33] . The lower chamber contained 10% FBS to attract the cells that were plated in medium containing 1% FBS. The assay was analysed after 24 h. Cell proliferation assays were performed with the Vybrant MTT cell proliferation assay kit (Invitrogen) according to supplier's instructions. Dilutions of each cell line, ranging from 1,000 to 5,000 cells per well, were plated in triplicates in 96-well plates and the cells were allowed to settle for 15 min at 37 °C ( t =0 h). 3-(4,5-dimethylthiazol-2-yl)-2,5-diphenyltetrazolium bromide (MTT) assay reagent was added to the cultures at the indicated time points and formazan formation was allowed to continue for 3 h. An exponential growth function y = A ×2 ( t / ôτ ) was fitted to the data. Fits with an adjusted R 2 value >0.95 were used to derive the doubling time ôτ for each cell line. Immunofluorescence microscopy Cells were fixed for 30 min at 21 °C with 4% formaldehyde in PBS, and permeabilized for 3 min with 0.1% Triton X-100 in PBS. Cells were stained with antibody to VCP (ab11433, Abcam) and Alexa Fluor 488 goat anti-mouse immunoglobulin G (Invitrogen) antibody diluted in PBS containing 1% bovine serum albumin. Confocal images spaced by 0.5 μm were taken with an Olympus FluoView 1,000 confocal laser scanning microscope using a PLAPON 60xO NA 1.42 objective. Average intensity z -projections were generated with ImageJ (URL: http://imagej.nih.gov/ij/ ). Preparation of S100 cytosolic extract A detergent-free cytosolic extract was prepared using hypotonic swelling, cell lysis using a Dounce-homogenizer and high speed centrifugation as described [34] . Partial purification of endogenous VCP from human cell lines HeLa wt or VCP-KMT-deficient cells were grown to ca. 70% confluence and lysed with 0.5% IGEPAL CA-630 in 20 mM Bis-Tris, pH 7.0 at 11 °C, 100 mM NaCl, 2 mM DTT and 1x complete protease inhibitor cocktail (Roche Applied Science). The lysate from ten 150 mm dishes per cell line was combined and centrifuged for 1 h at 4,600 g . The cleared lysate was loaded on a RESOURCE Q 6 ml column (GE Healthcare). After washing with 7.5 column volumes of buffer A (20 mM Bis-Tris, pH 7.0 at 11 °C, 100 mM NaCl, 2 mM DTT, 1 mM EDTA and 0.2 mM 4-(2-Aminoethyl) benzenesulfonyl fluoride hydrochloride (AEBSF)), bound proteins were eluted over 20 column volumes with a linear gradient from 0 to 50% Buffer B (20 mM Bis-Tris, pH 7.0 at 11 °C, 1 M NaCl, 2 mM DTT, 1 mM EDTA and 0.2 mM AEBSF). VCP containing fractions were identified by western blotting. The majority of VCP eluted between 28 and 32% B. These fractions were combined and concentrated to approximately 75 μl over Vivaspin 20 ultrafiltration units (molecular weight cutoff 100,000) (Sartorius-Stedim). The concentrate was applied to a Superose 6 10/300 GL column (GE Healthcare) using 150 mM NaCl, 20 mM Tris pH 8.0 at 11 °C, 1 mM MgCl 2 , 2 mM DTT as running buffer and 1 ml fractions were collected. All steps were performed on ice or in a cool cabinet at 11 °C. ATPase assays on cellular VCP The ATPase activity was assayed by adding 10 μl of each VCP-containing SEC-fraction (corresponding to 0.3–1 μg of protein) to 40 μl of 25 mM Tris pH 7.5, 10 mM MgCl 2 , 1 mM DTT and 150 μM ATP. After 1 h at 37 °C, the liberated phosphate was measured with Biomol Green assay reagent (Bio-Rad). Statistical analysis The independent two-sample Student's t -test (adjusted for unequal sample size for data shown in Fig. 5b ) was used for hypothesis testing, as a Shapiro-Wilk normality test showed no significant deviation from a normal distribution (alpha level 0.05) for all groups of interest, and equal variance of measurements can be assumed due to identical assay conditions. Tests were one-tailed for reduction of incorporation due to addition of inhibitor or mutation of key residues ( Fig. 6b ) and two-tailed in all other cases. The comparisons of interest were between means of groups and the alpha level was 0.05. How to cite this article: Kernstock, S. et al . Lysine methylation of VCP by a member of a novel human protein methyltransferase family. Nat. Commun. 3:1038 doi: 10.1038/ncomms2041 (2012).